Spontaneous tumour regression in keratoacanthomas is driven by Wnt/retinoic acid signalling cross-talk A fundamental goal in cancer biology is to identify the cells and signalling pathways that are keys to induce tumour regression. Here we use a spontaneously self-regressing tumour, cutaneous keratoacanthoma (KAs), to identify physiological mechanisms that drive tumour regression. By using a mouse model system that recapitulates the behaviour of human KAs, we show that self-regressing tumours shift their balance to a differentiation programme during regression. Furthermore, we demonstrate that developmental programs utilized for skin hair follicle regeneration, such as Wnt, are hijacked to sustain tumour growth and that the retinoic acid (RA) signalling pathway promotes tumour regression by inhibiting Wnt signalling. Finally, we find that RA signalling can induce regression of malignant tumours that do not normally spontaneously regress, such as squamous cell carcinomas. These findings provide new insights into the physiological mechanisms of tumour regression and suggest therapeutic strategies to induce tumour regression. Cancer does not generally spontaneously regress without treatment, although a clear rate of tumour regression is unknown given that internal organs cannot be closely monitored. However, solid tumours, such as melanoma, renal cell carcinoma and neuroblastoma, as well as non-solid tumours, such as lymphomas, occasionally do regress [1] , [2] , [3] . These regressing tumours represent an important model for identifying physiological mechanisms that drive tumour regression, providing potential insight for the development of targeted therapies for tumours that do not regress spontaneously. However, melanoma, renal cell carcinoma, neuroblastoma and lymphoma regress spontaneously rarely and unpredictably. In contrast, cutaneous KA, considered by many to be a behaviourally benign variant of squamous cell carcinoma (SCC), is defined as a self-regressing tumour. KA is characterized by rapid growth over a few weeks, followed by spontaneous resolution within the following few months [4] , [5] , [6] , [7] . While different hypotheses have been proposed to explain the mechanism of KA tumour regression [8] , [9] , [10] , to date we still lack a clear understanding of the signalling and cellular mechanisms that drive its spontaneous regression. The ability of KA to grow and regress is reminiscent of hair follicle cycling during physiological regeneration [11] . Hair follicles transition between growth phases, when the hair follicles expand in size, and regression phases, when most of the epithelial cells are eliminated leading to hair follicle shrinkage [12] , [13] . Hair follicle regeneration is driven by the orchestration of several well-characterized signalling pathways, including the Wnt pathway, which is a central signalling mechanism for the regeneration of several tissues. In the skin, Wnt signalling is activated at the onset of hair follicle growth through the action of Wnt ligands within the epithelium [12] , [14] , [15] , [16] . The binding of Wnt ligands to their receptors leads to stabilization and nuclear translocation of their effector β-catenin, which in turn activates the transcription of Wnt target genes such as Axin2, Cyclin D1 and Lef-1 (refs 17 , 18 , 19 , 20 ). Functionally, Wnt signalling is sufficient to induce hair follicle growth as shown by β-catenin gain of function studies [21] , [22] . Like Wnt, retinoic acid (RA) is another signalling pathway that plays an important role in tissue regeneration. In the skin, RA has been shown to repress proliferation and induce epidermal differentiation in mice [23] as well as regulate hair follicle regression in humans [24] . Developmental programs are often hijacked during cancer. Wnt signalling for instance has been implicated in several cancers, including colon and breast cancer [25] , [26] in addition to skin tumours such as SCC [27] , [28] . Malanchi et al. [29] have reported that Wnt signalling ablation impairs SCC tumour formation. Overall, these studies show how the Wnt signalling pathway is a dual key player that fuels both physiological tissue regeneration as well as tumour formation in several tissues. In the current study, we utilized a mouse model of self-regressing KA tumours. By using genetic lineage tracing experiments, we first show that hair follicle stem cell (HFSC) descendants contribute to tumour development and that these HFSC-derived cells actively contribute to different lineages within self-regressing tumours. We demonstrate that tumour regression is characterized by decreased proliferation, loss of HFSC descendants and increased differentiation. Strikingly, we demonstrate via an unbiased transcriptional approach that RA upregulation is an early event during the regression phase and that RA acts upstream of Wnt downregulation by inducing stromal Wnt inhibitors, which ultimately leads to tumour regression. Finally, we show that RA/Wnt signalling cross-talk is able to induce the regression of non -regressing tumours such as malignant SCC through Wnt inhibition and activation of differentiation programs. This suggests that differentiation and reduced proliferation are mechanisms utilized during spontaneous tumour regression and therefore provide the basis for therapy to eradicate tumours that do not regress spontaneously. HFSC-descendants contribute to self-regressing tumours In order to dissect the cellular mechanisms that sustain self-regressing KA tumour formation, we used a DMBA (7,12-dimethylbenz(a)anthracene) based chemical carcinogenetic protocol on mice [11] . Repeated applications of DMBA on the mouse back skin twice a week for up to 20 weeks led to a variety of skin epithelial tumours of which 40% were self-regressing KAs ( Supplementary Fig. 1a,b ). These epithelial self-regressing tumours mimicked the human variant ( Fig. 1a,b ; Supplementary Fig. 1c ) [4] . Reproducibly, DMBA withdrawal led to KA tumour regression within 6–8 weeks post-DMBA treatment therefore providing a robust model for studying the mechanisms that drive tumour regression. 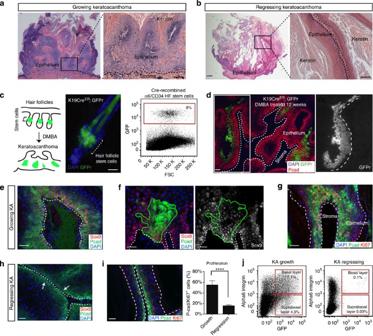Figure 1: Mouse KA tumours recapitulate human KAs and they originate from HFSC descendants. (a,b) Hematoxylin and eosin staining shows mouse KA in the growth phase and the regression phase (scale bar, 100 μm for pictures on the left, and 50 μm for pictures on the right). (c) Schematic representation of the genetic lineage tracing approach utilized for labelling the HFSCs. Representative image of a hair follicle from tamoxifen-treatedKrt19CreER;Rosa26 mTmGFPmice. The fluorescent reporter (GFPr, in green) labels the stem cells and the progeny. Dotted bracket indicates the location of the stem cells within the hair follicle (scale bar, 20 μm). Flow cytometry analysis of GFP+cells in the HFSC compartment prior to DMBA treatment (n=3). (d) DMBA was applied to tamoxifen-treatedK19CreER;Rosa26mTmGFPmice. Twelve weeks post-DMBA treatment, GFP+hair follicle descendant cells were found in the epithelium of KA tumours, as shown by GFP (green) co-localization with P-cadherin (red) (n=18, scale bar, 50 μm). (e,h) Sox9 staining in KA tumours sections during growth and regression phases (n=3, scale bar, 50 μm). (f) Immunofluorescence staining for Sox9 showing co-localization with the HFSCs-derived cells (HFSCs, green) after Cre recombination tamoxifen mediated. Continuous green lines identify the HFSC descendants (scale bar, 50 μm). (g,i) Immunofluorescence staining for the proliferation marker Ki67 in KAs tumours during growth and regression phase shows reduction in the number of Ki67+(red) and P-cadherin+(green) cells during regression (scale bar, 50 μm). Cell proliferation has been quantified in KA during growth or regression (n=4). Data are represented as mean±s.d., ****<0.001 obtained by unpairedt-test analysis. (j) Representative flow cytometry analysis of HFSC-derived GFP+cells during KA growth and regression (n=7 andn=8, respectively). In all the pictures, dotted lines indicate the tumour/stroma interface. In all the immunofluorescence experiments performed, nuclei are marked in blue with DAPI. Figure 1: Mouse KA tumours recapitulate human KAs and they originate from HFSC descendants. ( a , b ) Hematoxylin and eosin staining shows mouse KA in the growth phase and the regression phase (scale bar, 100 μm for pictures on the left, and 50 μm for pictures on the right). ( c ) Schematic representation of the genetic lineage tracing approach utilized for labelling the HFSCs. Representative image of a hair follicle from tamoxifen-treated Krt19Cre ER ; Rosa26 mTmGFP mice. The fluorescent reporter (GFPr, in green) labels the stem cells and the progeny. Dotted bracket indicates the location of the stem cells within the hair follicle (scale bar, 20 μm). Flow cytometry analysis of GFP + cells in the HFSC compartment prior to DMBA treatment ( n =3). ( d ) DMBA was applied to tamoxifen-treated K19Cre ER ; Rosa26mTmGFP mice. Twelve weeks post-DMBA treatment, GFP + hair follicle descendant cells were found in the epithelium of KA tumours, as shown by GFP (green) co-localization with P-cadherin (red) ( n =18, scale bar, 50 μm). ( e , h ) Sox9 staining in KA tumours sections during growth and regression phases ( n =3, scale bar, 50 μm). ( f ) Immunofluorescence staining for Sox9 showing co-localization with the HFSCs-derived cells (HFSCs, green) after Cre recombination tamoxifen mediated. Continuous green lines identify the HFSC descendants (scale bar, 50 μm). ( g , i ) Immunofluorescence staining for the proliferation marker Ki67 in KAs tumours during growth and regression phase shows reduction in the number of Ki67 + (red) and P-cadherin + (green) cells during regression (scale bar, 50 μm). Cell proliferation has been quantified in KA during growth or regression ( n =4). Data are represented as mean±s.d., ****<0.001 obtained by unpaired t -test analysis. ( j ) Representative flow cytometry analysis of HFSC-derived GFP + cells during KA growth and regression ( n =7 and n =8, respectively). In all the pictures, dotted lines indicate the tumour/stroma interface. In all the immunofluorescence experiments performed, nuclei are marked in blue with DAPI. Full size image The ability of KA tumours to grow and regress is reminiscent of the ability of hair follicles to cycle through growth and regression phases. Thus, we hypothesized that HFSCs/HFSC descendants could fuel self-regressing tumours ( Fig. 1c ). To test this hypothesis, we permanently labelled HFSCs by utilizing mice carrying the tamoxifen-inducible Keratin 19Cre ER -along with a green fluorescent protein ( GFP ) Cre-reporter (GFPr) [30] ( Fig. 1c and Supplementary Fig. 1d ). Upon subsequent DMBA treatment, induced tumours were collected, sectioned and stained for anti-GFP. Immunofluorescence analysis showed that GFP + HFSC-derived cells were found within several regions of self-regressing tumours ( Fig. 1d ), despite the initial low labelling efficiency of HFSCs. Strikingly, the number of stem cell-derived GFP + cells was dramatically reduced in 6-week regressing tumours by fluorescence-activated cell sorting (FACS) ( Fig. 1j and Supplementary Fig. 2a,b ). Given our observation that HFSCs/HFSC descendants are present within regressing tumours, we asked whether HFSC markers were also retained within the tumours. Immunofluorescence for a variety of stem cell markers showed that several, such as CD34, Krt15 and Lgr5, were not expressed. In contrast, we found that Sox9—a Wnt target gene and a key regulator of HFSCs during hair follicle regeneration—was still expressed, along with other undifferentiated adhesion molecules, such as P-cadherin, α6 and β4 integrin ( Figs 1e and 2c ). This pattern of expression was also present within the HFSC-derived cells as shown by co-localization of Sox9 with GFP in the Krt19Cre ER ; GFPr mice ( Fig. 1f ). However, and similarly to the lineage tracing experiments, Sox9 levels were dramatically reduced during the tumour regression phase ( Fig. 1h ). Consistent with these findings, self-regressing tumours were highly proliferative during the growth phase, but displayed a dramatic decrease of proliferative cells during the regression phase (Ki67 proliferative marker and hair follicle epithelial marker P-cadherin— Fig. 1g,i ). All together, these findings demonstrate that HFSC/HFSC-descendant cells contribute to the development of self-regressing skin tumours and suggest that the regression phase is characterized by the shrinkage of the undifferentiated/proliferative pool. 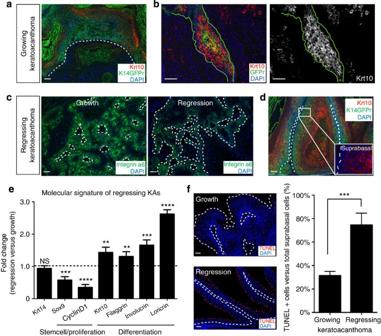Figure 2: Increased differentiation characterize KA tumour regression. (a,d) KAs tumours show different expression of differentiation markers Krt10 (scale bar, 50 μm). (b) HFSC descendants within KA tumours (green labelling) show co-localization with Krt10. Continuous green line identifies the HFSC descendants (scale bar, 50 μm). (c) Immunofluorescence staining showing maintained expression of integrin α6 in growth and regression phase (scale bar, 50 μm). (e) qRT–PCR from whole KA tumour RNA in the regression phase. Krt14 expression levels are used as control. The comparison has been conducted by using the ΔΔCT method and normalized to Glyceraldehyde-3-phosphate dehydrogenase transcript. Dotted line represents the normalized expression level of each transcript analysed during tumour growth. Data are represented as mean±s.d. (n=4) (**<0.05, ***<0.001, ****<0.005 obtained by unpairedt-test statistical analysis). (f) Immunofluorescence staining for TUNEL and its relative quantification (KA regression versus KA growth) (n=4, ***<0.001, obtained by unpairedt-test statistical analysis) (scale bar, 50 μm). In all the pictures, dotted lines indicate the tumour/stroma interface. Nuclei are marked in blue with DAPI. Figure 2: Increased differentiation characterize KA tumour regression. ( a , d ) KAs tumours show different expression of differentiation markers Krt10 (scale bar, 50 μm). ( b ) HFSC descendants within KA tumours (green labelling) show co-localization with Krt10. Continuous green line identifies the HFSC descendants (scale bar, 50 μm). ( c ) Immunofluorescence staining showing maintained expression of integrin α6 in growth and regression phase (scale bar, 50 μm). ( e ) qRT–PCR from whole KA tumour RNA in the regression phase. Krt14 expression levels are used as control. The comparison has been conducted by using the ΔΔCT method and normalized to Glyceraldehyde-3-phosphate dehydrogenase transcript. Dotted line represents the normalized expression level of each transcript analysed during tumour growth. Data are represented as mean±s.d. ( n =4) (**<0.05, ***<0.001, ****<0.005 obtained by unpaired t -test statistical analysis). ( f ) Immunofluorescence staining for TUNEL and its relative quantification (KA regression versus KA growth) ( n =4, ***<0.001, obtained by unpaired t -test statistical analysis) (scale bar, 50 μm). In all the pictures, dotted lines indicate the tumour/stroma interface. Nuclei are marked in blue with DAPI. Full size image KA tumours activate differentiation during regression We wanted to investigate whether the loss of undifferentiated cells observed during the regression phase was driven by cell death or differentiation mechanisms in addition to decreased proliferation. To address whether apoptosis takes place during regression, we stained for activated cleaved Caspase 3 antibody. Immunofluorescence analyses showed very few activated cleaved Caspase 3 + cells during regression and it showed no difference when compared with the tumour growth phase ( Supplementary Fig. 3a,b ). Next, we assayed for a variety of skin differentiation markers. While hair follicle differentiation markers failed to be detected, markers of epidermal differentiation were expressed in the self-regressing tumour cells, specifically Krt10 and TUNEL [31] ( Fig. 2a,f and Supplementary Fig. 4a,b ). Surprisingly, we found that GFP + HFSC descendants within the tumours were positive for such epidermal differentiation markers ( Fig. 2b ; Supplementary Fig. 4c ). These results suggest that HFSC-derived GFP + cells have the ability to change their molecular signature to adapt and be functionally active within the tumour. Finally, we addressed whether and how the above-characterized expression pattern would change during the tumour regression phase. We found that the expression of differentiation markers was increased in the regression phase versus growth phase by immunofluorescence and quantitative real time polymerase chain reaction (qRT–PCR) ( Fig. 2d,e ). All together, these findings demonstrate that HFSC-descendant cells recruited in self-regressing tumours change their signature to adapt to the tumour environment and that spontaneous tumour regression is driven by an increase of the differentiation programme. Wnt signalling is differentially regulated in KA tumours In order to identify the molecular mechanisms that are responsible for KA self-regression, we evaluated stem cell signalling pathways that have been shown to play a crucial role in tissue regeneration. Among the several signalling pathways that we screened by qRT–PCR, Wnt components stood out as the most differentially expressed between the regression and growth phase of KA tumours (data not shown). We found that during the growth phase more than 80% of tumour epithelial cells displayed nuclear β-catenin, a hallmark of activated Wnt pathway. In contrast, only 17% of nuclear β-catenin + cells were found during the regression phase ( Fig. 3a,b ). Similarly, self-regressing tumours generated in Wnt reporter mice [32] show that the large majority of epithelial cells activated the Wnt reporter ( Supplementary Fig. 5a,b ). These combined evidences suggest that Wnt pathway is active during the growth phase compared with the regressing phase. 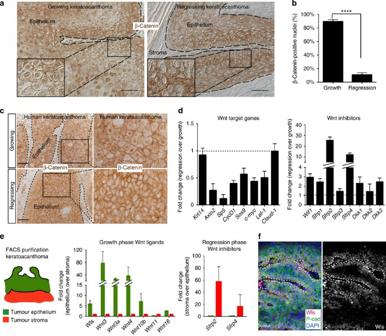Figure 3: Wnt signalling is differentially regulated in growing and regressing KAs. (a) β-Catenin immunohistochemistry on growing and regressing KAs (see also insets) (scale bar, 50 μm). (b) Quantification for nuclear β-catenin fraction in KAs confirmed a statistically significant reduction of nuclear β-catenin-positive cells in regressing KAs. Data are represented as mean±s.d. (n=4) (****<0.001 obtained by unpairedt-test statistical analysis). (c) Wnt signalling is differentially expressed in human KAs. Nuclear β-catenin immunohistochemistry shows Wnt activation in growing KAs, while absence of nuclear β-catenin indicates Wnt downregulation in human regressing KAs (scale bar, 50 μm). (d) qRT–PCR analysis of Wnt target genes and inhibitors in growing and regressing KAs. The comparison has been conducted by using the ΔΔCT method and normalized to glyceraldehyde-3-phosphate dehydrogenase (GAPDH) transcript. Dotted line represents the normalized expression level of each transcript analysed during tumour growth. Data are represented as mean±s.d. (n=4). (e)Krt14Cre;Rosa26mTmGFPmice have been used for FACS sorting epithelial and stromal cells from KA tumours in growth and regression phase. GFP (green) marks all the KA epithelial cells, while tomato (red) labels the tumoural stroma. Center panel: qRT–PCR expression analysis of the Wnt ligands in growing KAs comparing epithelium versus stroma. Right panel: qRT–PCR expression analysis of the Wnt inhibitors in regressing KAs comparing stroma versus epithelium. Both comparisons have been conducted by using the ΔΔCT method and normalized to GAPDH transcript. Data are represented as mean±s.d. (n=3). (f) Immunofluorescence staining for Wntless (Wls) and P-cadherin shows expression in KA tumoural epithelium (scale bar, 50 μm). In all the pictures, dotted lines delineate the tumour/stroma interface. In all the immunofluorescence experiments performed, nuclei are marked in blue with DAPI. Figure 3: Wnt signalling is differentially regulated in growing and regressing KAs. ( a ) β-Catenin immunohistochemistry on growing and regressing KAs (see also insets) (scale bar, 50 μm). ( b ) Quantification for nuclear β-catenin fraction in KAs confirmed a statistically significant reduction of nuclear β-catenin-positive cells in regressing KAs. Data are represented as mean±s.d. ( n =4) (****<0.001 obtained by unpaired t -test statistical analysis). ( c ) Wnt signalling is differentially expressed in human KAs. Nuclear β-catenin immunohistochemistry shows Wnt activation in growing KAs, while absence of nuclear β-catenin indicates Wnt downregulation in human regressing KAs (scale bar, 50 μm). ( d ) qRT–PCR analysis of Wnt target genes and inhibitors in growing and regressing KAs. The comparison has been conducted by using the ΔΔCT method and normalized to glyceraldehyde-3-phosphate dehydrogenase (GAPDH) transcript. Dotted line represents the normalized expression level of each transcript analysed during tumour growth. Data are represented as mean±s.d. ( n =4). ( e ) Krt14Cre ; Rosa26mTmGFP mice have been used for FACS sorting epithelial and stromal cells from KA tumours in growth and regression phase. GFP (green) marks all the KA epithelial cells, while tomato (red) labels the tumoural stroma. Center panel: qRT–PCR expression analysis of the Wnt ligands in growing KAs comparing epithelium versus stroma. Right panel: qRT–PCR expression analysis of the Wnt inhibitors in regressing KAs comparing stroma versus epithelium. Both comparisons have been conducted by using the ΔΔCT method and normalized to GAPDH transcript. Data are represented as mean±s.d. ( n =3). ( f ) Immunofluorescence staining for Wntless (Wls) and P-cadherin shows expression in KA tumoural epithelium (scale bar, 50 μm). In all the pictures, dotted lines delineate the tumour/stroma interface. In all the immunofluorescence experiments performed, nuclei are marked in blue with DAPI. Full size image To test whether Wnt dynamic regulation occurs in human self-regressing tumours, we performed β-catenin immunohistochemistry on sections of human KA tumours both in growth and regression phases. Similarly to the mouse self-regressing tumour behaviour, nuclear β-catenin was observed in the majority of the epithelium of growing human KAs, while β-catenin primarily stained the cell membrane in regressing human KAs ( Fig. 3c ). Thus, the observation that Wnt downregulation was conserved in the human tumour regression phase considerably raised the relevance of these results and encouraged us to pursue the significance of these findings in our mouse model for self-regressing tumours. If Wnt pathway is downregulated during the regression phase, Wnt target genes ought to be downregulated. Wnt target genes, such as Axin2, Sox9, Cyclin D1 and Lef1 , were downregulated in the regression phase versus the growth phase by qRT–PCR ( Fig. 3d ). We hypothesized that Wnt downregulation might be triggered by Wnt inhibitor upregulation. Wnt inhibitors are a small group of soluble proteins that antagonize Wnt activation by preventing ligand-receptor activation or inhibiting Wnt receptor maturation [33] . When we analysed Wnt inhibitor expression by qRT–PCR, we found that regressing KAs displayed high levels of several Wnt inhibitors, with Sfrp2 and Sfrp4 being the most predominantly expressed ( Fig. 3d ). All together, these data demonstrate that the Wnt signalling pathway is downregulated in KAs during regression presumably via upregulation of Wnt inhibitors. To begin to shed light on the mechanisms of tumour regression, we sought to identify the source of both Wnt ligands and inhibitors during the growth and regression phases. During hair follicle development and regeneration, Wnt ligands are mostly produced by the epithelium and Wnt inhibitors by the stroma [34] . Thus, we have used mice carrying Keratin 14Cre; Tomato-GFPr alleles to FACS purify epithelial (GFP + /Tomato − ) and stromal (GFP − /Tomato + ) populations from the self-regressing tumours (cartoon in Fig. 3e ; Supplementary Fig. 5c ). qRT–PCR analysis of the FACS-purified populations showed that most of the Wnt ligands, such as Wnt3, Wnt3a, Wnt4 and Wnt10b , along with Wntless (Wls) , a gene required for Wnt ligand secretion [16] , were highly upregulated in the epithelial cells during the growth phase ( Fig. 3e,f and Supplementary Fig. 5d,e ). Conversely, Wnt inhibitor transcripts, predominantly Sfrp2 and Sfrp4 , were upregulated in the stromal cells when compared with epithelial cells during the regression phase ( Fig. 3e and Supplementary Fig. 5d ). All together, these data show that Wnt is differentially regulated in the two different KA tumour stages and that communication between the epithelium and the stromal component of KA tumours may play an important role in regulating Wnt signalling similarly to what is observed during development. Wnt inhibition is sufficient to induce tumour regression We have thus shown that Wnt signalling is downregulated in regressing KAs. We therefore reasoned that if Wnt downregulation is sufficient to induce KA regression, forced inhibition of the Wnt pathway during the growth phase would trigger precocious tumour regression ( Fig. 4a ). In order to test this hypothesis, we injected growing KA tumours with either the Wnt inhibitor IWP2 or vehicle while continuing DMBA treatment. IWP2 is a compound that prevents Wnt ligand palmitoylation by the enzyme porcupine, resulting in impaired Wnt ligand secretion [35] . As early as 2 days after treatment, a dramatic reduction of more than five fold in the number of nuclear β-catenin + cells was observed in the IWP2 versus vehicle-injected tumours, which confirms the efficacy of the treatment ( Fig. 4b,c ). Consistent with the lack of nuclear β-catenin, Wnt target genes Axin2, Cyclin D1, Sox9 and Lef1 were downregulated 2 days post treatment by qRT–PCR ( Fig. 4d —black bars). 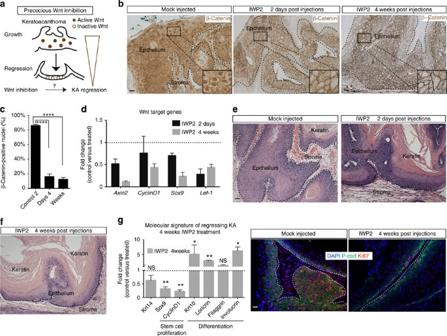Figure 4: Wnt inhibition is sufficient to induce KA regression. (a) Schematic model for Wnt inhibition as trigger for KA regression. (b,c) β-Catenin immunohistochemistry on IWP2-treated tumours versus mock-injected tumours (scale bar, 50 μm). Nuclear β-catenin quantification of the number of nuclear β-catenin+cells at the 2 days and 4 weeks time points of IWP2-treated tumours (83%±2 versus 17%±3 and 15%±2, respectively). Data are represented as mean±s.d. (n=4) (****<0.001 obtained by unpairedt-test statistical analysis) (scale bar, 50 μm). (d) qRT–PCR analysis on IWP2- versus mock-injected KA tumours of Wnt target genes at both 2 days and 4 weeks post injections. Dotted line represents the normalized expression level of each transcript analysed during tumour growth. Data are represented as mean±s.d. (n=4). (e) Hematoxylin and eosin staining performed on IWP2 and PBS-injected tumours at 2 days and 4 weeks post injections (scale bar, 50 μm). (f) qRT–PCR for proliferation and terminal differentiation markers in IWP2-injected KAs. Dotted line represents the normalized expression level of each gene analysed during tumour growth. Data are represented as mean±s.d. (n=4) (**<0.005, *<0.01, obtained by unpairedt-test statistical analysis). (g) Ki67 (red) and P-cadherin (green) immunofluorescence staining on IWP2- and mock-injected tumours. DAPI (blue) labels all the nuclei (scale bar, 50 μm). Dotted lines delineate the tumour/stroma interface. Figure 4: Wnt inhibition is sufficient to induce KA regression. ( a ) Schematic model for Wnt inhibition as trigger for KA regression. ( b , c ) β-Catenin immunohistochemistry on IWP2-treated tumours versus mock-injected tumours (scale bar, 50 μm). Nuclear β-catenin quantification of the number of nuclear β-catenin + cells at the 2 days and 4 weeks time points of IWP2-treated tumours (83%±2 versus 17%±3 and 15%±2, respectively). Data are represented as mean±s.d. ( n =4) (****<0.001 obtained by unpaired t -test statistical analysis) (scale bar, 50 μm). ( d ) qRT–PCR analysis on IWP2- versus mock-injected KA tumours of Wnt target genes at both 2 days and 4 weeks post injections. Dotted line represents the normalized expression level of each transcript analysed during tumour growth. Data are represented as mean±s.d. ( n =4). ( e ) Hematoxylin and eosin staining performed on IWP2 and PBS-injected tumours at 2 days and 4 weeks post injections (scale bar, 50 μm). ( f ) qRT–PCR for proliferation and terminal differentiation markers in IWP2-injected KAs. Dotted line represents the normalized expression level of each gene analysed during tumour growth. Data are represented as mean±s.d. ( n =4) (**<0.005, *<0.01, obtained by unpaired t -test statistical analysis). ( g ) Ki67 (red) and P-cadherin (green) immunofluorescence staining on IWP2- and mock-injected tumours. DAPI (blue) labels all the nuclei (scale bar, 50 μm). Dotted lines delineate the tumour/stroma interface. Full size image To test whether Wnt inhibition is sufficient to induce tumour regression, we continued to treat the tumours with DMBA and analysed them after 4 weeks from the last IWP2 injection. Strikingly, tumours injected with IWP2 entered precocious regression whereas vehicle-treated tumours were still in growth as shown by histological, immunofluorescence and qRT analysis ( Fig. 4e,g ). All together, these findings identify Wnt inhibition as a key molecular mechanism sufficient to induce precocious KA tumour regression. To address whether Wnt inhibition is required for tumour self-regression, we employed an inducible genetic mouse model to stabilize β-catenin and constitutively activate the Wnt pathway within the epithelial cells ( Fig. 5a ). Mice carrying triple alleles Keratin14Cre ER ;GFPr; β -catn flox(Ex3)/+ (refs 36 , 37 ) or Keratin14Cre ER ;GFPr littermates were induced with tamoxifen to activated the Cre at 16 weeks of DMBA treatment. In the case of the mutant mice, Cre activation resulted in β-catenin exon 3 removal, which in turn leads to β-catenin stabilization. After tamoxifen induction, mutants and control mouse littermates were then kept for six weeks in the absence of DMBA. Strikingly, our results showed that β-catenin stabilization maintained KA tumours in the growth phase while control littermate KAs had entered the regression phase ( Fig. 5b–d ). To verify that the mutant tumour behaviour was due to β-catenin activation, we performed β-catenin immunohistochemistry. As expected, a large number of nuclear β-catenin + cells were detected in the Keratin14Cre ER ;GFPr; β -catn flox(Ex3)/+ mice whereas mostly membrane-bound β-catenin was observed in the control Keratin14Cre ER ;GFPr littermates by immunohistochemistry ( Fig. 5c,d ). Taken together, these findings demonstrate that Wnt inhibition is sufficient and necessary to induce spontaneous tumour regression. 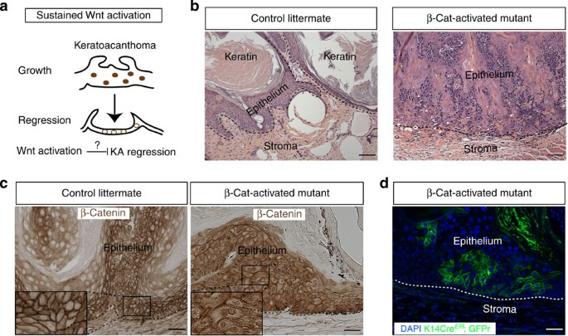Figure 5: Wnt inhibition is required to induce KA regression. (a) Schematic representation of the role of constitutive Wnt activation to inhibit KA tumour regression. (b) Histological analysis ofK14CreER;Rosa26mTmGFP; β-catnflox(Ex3)/+and control littermates showing that Wnt constitutive activation inhibits tumour regression (n=5 for control littermates and mutant) (scale bar, 50 μm). (c) β-Catenin immunohistochemistry onK14CreER;Rosa26mTmGFP;β-catnflox(Ex3)/+and control littermates shows nuclear β-catenin localization in the mutant tumours in comparison with the control ones where β-catenin is expressed in the membrane (scale bar, 50 μm). (d) KA tumour fromK14CreER;Rosa26mTmGFP; β-catnflox(Ex3)/+mice stained with an anti-GFP antibody showing the localization of β-catenin-mutant cells within KA tumours (scale bar, 50 μm). Nuclei are labelled with DAPI (blue). Dotted lines delineate the tumour/stroma interface. Figure 5: Wnt inhibition is required to induce KA regression. ( a ) Schematic representation of the role of constitutive Wnt activation to inhibit KA tumour regression. ( b ) Histological analysis of K14Cre ER ; Rosa26mTmGFP ; β -catn flox(Ex3)/+ and control littermates showing that Wnt constitutive activation inhibits tumour regression ( n =5 for control littermates and mutant) (scale bar, 50 μm). ( c ) β-Catenin immunohistochemistry on K14Cre ER ; Rosa26mTmGFP; β -catn flox(Ex3)/+ and control littermates shows nuclear β-catenin localization in the mutant tumours in comparison with the control ones where β-catenin is expressed in the membrane (scale bar, 50 μm). ( d ) KA tumour from K14Cre ER ; Rosa26mTmGFP ; β -catn flox(Ex3)/+ mice stained with an anti-GFP antibody showing the localization of β-catenin-mutant cells within KA tumours (scale bar, 50 μm). Nuclei are labelled with DAPI (blue). Dotted lines delineate the tumour/stroma interface. Full size image RA activation and Wnt downregulation induce tumour regression Wnt downregulation was observed in advanced stages of tumour regression at 6 weeks post-DMBA treatment. Thus, we asked which signalling pathways could act initially and be responsible for Wnt downregulation. In order to address this question, we used an unbiased approach and performed RNA sequencing to compare the transcriptional profile of epithelial cells of KA tumours at 0 and 1 week post-DMBA treatment. We found that a total number of 107 genes were differentially regulated between the time points analysed ( Supplementary Table 1 ). Among others, we found that the RA signalling pathway stood out as RA-related transcripts Crabp1, Fam5C (Brinp3) and Cyp26b1 were upregulated at 1 week post DMBA ( Fig. 6a in red). During mouse development and hair follicle regeneration, the RA pathway has been shown to inhibit Wnt pathway [17] , [38] . qRT–PCR of RA-related transcripts both in the epithelial population only as well as in whole tumour ( Supplementary Fig. 6a ) shows that RA activation is an early event during KA tumour regression. If RA acts during the regression phase by downregulating Wnt, then RA upregulation ought to occur prior to Wnt downregulation during KA regression. To test this hypothesis, we first treated wild-type keratinocytes with RA in vitro . Consistent with our model, we found that RA-treated keratinocytes induced not only upregulation of Wnt inhibitors Sfrp2 and Sfrp4 but also promoted downregulation of Wnt target genes by qRT–PCR ( Supplementary Fig. 6b ). This finding establishes a link between RA upregulation and Wnt downregulation in skin epithelial cells. 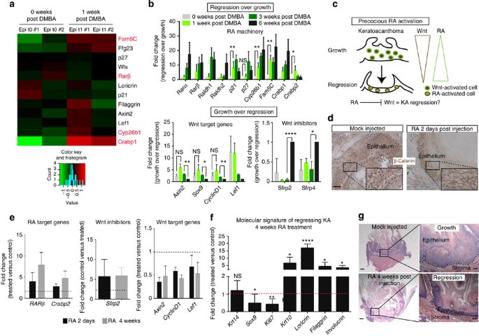Figure 6: RA downregulates Wnt and promote KA tumour regression. (a) RNA sequencing heatmap showing a subset of genes differentially expressed between tumour in growth (0 weeks post DMBA) and early regression (1 week post DMBA). The colour coded values are mean centred log10(CPM+1). CPM (count per million): number of reads mapped to a gene for each million reads mapped to any genes. (b) qRT–PCR analysis of RA and Wnt signalling pathway on 0, 1, 3 and 6 weeks post-DMBA treatment. All the values are normalized to the 6-week post-DMBA time point. Data are represented as mean±s.d. (n=3 for each time point) (**<0.01, *<0.05, obtained by unpairedt-test statistical analysis). (c) Schematic representation that represents RA/Wnt cross-talk in regressing KAs. (d) Immunohistochemistry analysis for nuclear β-catenin+cells in RA and mock-injected KAs (scale bar, 50 μm). (e) qRT–PCR analysis on RA and mock-injected KA tumours at 2 days and 4 weeks after last injection (n=5). (f) qRT–PCR analysis of proliferation and differentiation genes in RA and vehicle-injected KA tumours. RA versus mock-injected tumours comparison has been conducted by using the ΔΔCT method and normalized to glyceraldehyde-3-phosphate dehydrogenase transcript. Data are represented as mean±s.d. (n=5). Dotted line represents the normalized expression level of each gene analysed for the experiment (*<0.05, **<0.01, ****<0.001, obtained by unpairedt-test statistical analysis). (g) Hematoxylin and eosin staining performed on RA and mock-injected tumours at 4 weeks post injection (scale bar, 200 μm for the pictures on the left and 50 μm for the pictures on the right). Dotted lines delineate the tumour/stroma interface. Figure 6: RA downregulates Wnt and promote KA tumour regression. ( a ) RNA sequencing heatmap showing a subset of genes differentially expressed between tumour in growth (0 weeks post DMBA) and early regression (1 week post DMBA). The colour coded values are mean centred log10(CPM+1). CPM (count per million): number of reads mapped to a gene for each million reads mapped to any genes. ( b ) qRT–PCR analysis of RA and Wnt signalling pathway on 0, 1, 3 and 6 weeks post-DMBA treatment. All the values are normalized to the 6-week post-DMBA time point. Data are represented as mean±s.d. ( n =3 for each time point) (**<0.01, *<0.05, obtained by unpaired t -test statistical analysis). ( c ) Schematic representation that represents RA/Wnt cross-talk in regressing KAs. ( d ) Immunohistochemistry analysis for nuclear β-catenin + cells in RA and mock-injected KAs (scale bar, 50 μm). ( e ) qRT–PCR analysis on RA and mock-injected KA tumours at 2 days and 4 weeks after last injection ( n =5). ( f ) qRT–PCR analysis of proliferation and differentiation genes in RA and vehicle-injected KA tumours. RA versus mock-injected tumours comparison has been conducted by using the ΔΔCT method and normalized to glyceraldehyde-3-phosphate dehydrogenase transcript. Data are represented as mean±s.d. ( n =5). Dotted line represents the normalized expression level of each gene analysed for the experiment (*<0.05, **<0.01, ****<0.001, obtained by unpaired t- test statistical analysis). ( g ) Hematoxylin and eosin staining performed on RA and mock-injected tumours at 4 weeks post injection (scale bar, 200 μm for the pictures on the left and 50 μm for the pictures on the right). Dotted lines delineate the tumour/stroma interface. Full size image Next, we tested whether RA signalling activation is associated with Wnt inhibition during advanced tumour regression. Thus, we performed a time course experiment during tumour regression and looked at the RA and Wnt components at 0, 1, 3 and 6 weeks post-DMBA treatment by qRT–PCR. We confirmed that the RA signalling machinery was activated as early as 1 week post-DMBA treatment, although the highest upregulation occurred later at 3 and 6 weeks ( Fig. 6a,b ). In contrast, most of the Wnt target genes, such as Axin2 and Lef-1 , were still upregulated at the 3-week time point but became downregulated at 6 weeks post-DMBA treatment when Wnt inhibitors started to be upregulated. Overall, these data indicate that the RA signalling pathway activation occurs prior to Wnt inhibition during early stages of KA regression and that a certain threshold of RA upregulation may be necessary to trigger Wnt inhibition. In order to test whether RA is able to induce Wnt downregulation in vivo, we injected KA tumours with RA ( Fig. 6c ). As early as 2 days after the last RA injection, KAs displayed a dramatic reduction in the number of nuclear β-catenin + cells in comparison with vehicle-injected tumours ( Fig. 6d ). In addition, upregulation of Wnt inhibitor Sfrp2 and downregulation of several Wnt target genes, including Axin2 and Sox9 , was observed by qRT–PCR ( Fig. 6e —black bars). To test if RA treatment induced KA precocious regression, we waited for 4 weeks post RA injection while DMBA treatment was continued. Strikingly, we found that RA-treated tumours had entered the regression phase by activating differentiation programs, while the vehicle-injected tumours were still growing ( Fig. 6f,g ). If β-catenin acts downstream of RA activation, we reasoned that constitutive activation of Wnt signalling would impair RA efficacy. To test this hypothesis, we treated KA tumours derived from Keratin14Cre ER ;GFPr; β -catn flox(Ex3)/+ mice with RA. We found that Wnt-stabilized KA tumours were not affected by RA treatment, as shown by tumour histology and nuclear β-catenin staining of both RA-treated and vehicle-treated KAs ( Supplementary Fig. 7 ). All together, these findings demonstrate that the RA signalling pathway is sufficient to induce Wnt downregulation in KA tumours as well as precocious regression of KAs via inhibition of Wnt pathway. RA activation leads to Wnt inhibition and SCC regression If RA/Wnt signalling is able to induce physiological tumour regression, we reasoned that the same cross-talk could induce the regression of skin tumours that do not spontaneously regress. To address this question, we used skin SCC as a model system. SCC tumours start to develop on the mouse back skin after 20 weeks of DMBA treatment. We first compared the levels of RA machinery in growing KAs, regressing KAs and SCCs. We found that RA signalling levels were lower in SCC tumours in comparison with regressing KA, as shown by qRT–PCR analysis for RA machinery ( Fig. 7a ). Consistent with these findings, Wnt ligands and inhibitors level in SCCs were comparable with KA in growth ( Supplementary Fig. 8a ). To test if RA dynamic regulation occurs in human skin tumour, we stained SCC tumours, as well as growing and regressing KAs for the RA-associated protein Crabp2. Crabp2 translocates from the cytoplasm to the nucleus to activate RA pathway. Strikingly, we found that Crabp2 was nuclear in regressing human KAs while it was predominantly cytoplasmic in growing KA and SCC human tumours ( Fig. 7b ). These findings prompted us to ask whether forced expression of RA signalling could result in regression of SCC tumours ( Supplementary Fig. 8b ). To address this question, we have injected RA or mock to SCCs for 7 consecutive days and waited for 4 weeks. RA activation was confirmed by qRT–PCR analysis post RA treatment and by nuclear staining for Crabp2 ( Supplementary Fig. 8b,c ). At 4-week post treatment, we found that RA injection led to regression of both KAs/papillomas (black) and SCCs (red) as quantified over time by macroscopic measurements ( Fig. 7c ). qRT–PCR analysis of RA and mock-injected SCC tumours showed that tumour regression was driven by loss of proliferation and increased differentiation programs ( Fig. 7d ). In addition, qRT–PCR analysis of Wnt target genes, as well as immunohistochemistry for Sox9 and β-catenin, showed that RA treatment induced Wnt inhibition in regressing SCCs ( Fig. 7e,f and Supplementary Fig. 8d ). 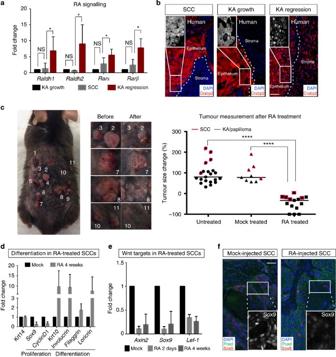Figure 7: RA induces SCC tumour regression. (a) RNA levels of RA in mouse SCC, KA in growth and regression. Data are represented as mean±s.d. (n=5 for each tumour analysed, *<0.05 obtained by unpairedt-test statistical analysis). (b) Immunofluorescence staining for Crabp2 in human SCC tumours, growing and regressing KAs (n=2 for each tumour). (c, left and central panel) Mouse treated with RA showing skin tumour regression (including SCC in the micrographs). (right panel) % of tumour growth rate by comparing untreated, mock-treated and RA-treated skin tumours at the fourth week post RA treatment. Red boxes indicate SCC tumours that have been diagnosed for each category, black box indicate KA and papilloma tumours (****<0.001 obtained by unpairedt-test statistical analysis). (d) qRT–PCR analysis for proliferation and differentiation genes in mock- and RA-injected SCC tumours. RA- versus mock-injected tumour comparison has been conducted by using the ΔΔCT method and normalized to glyceraldehyde-3-phosphate dehydrogenase (GAPDH) transcript. Data are represented as mean±s.d. (n=7). (e) qRT–PCR analysis for Wnt target genes in mock- and RA-injected SCC tumours. RA versus mock-injected tumours comparison has been conducted by using the ΔΔCT method and normalized to GAPDH transcript. Data are represented as mean±s.d. (n=5). (f) Immunofluorescence staining for Sox9 in mock- and RA-injected SCC tumours (scale bar, 50 μm). Figure 7: RA induces SCC tumour regression. ( a ) RNA levels of RA in mouse SCC, KA in growth and regression. Data are represented as mean±s.d. ( n =5 for each tumour analysed, *<0.05 obtained by unpaired t- test statistical analysis). ( b ) Immunofluorescence staining for Crabp2 in human SCC tumours, growing and regressing KAs ( n =2 for each tumour). ( c , left and central panel) Mouse treated with RA showing skin tumour regression (including SCC in the micrographs). (right panel) % of tumour growth rate by comparing untreated, mock-treated and RA-treated skin tumours at the fourth week post RA treatment. Red boxes indicate SCC tumours that have been diagnosed for each category, black box indicate KA and papilloma tumours (****<0.001 obtained by unpaired t -test statistical analysis). ( d ) qRT–PCR analysis for proliferation and differentiation genes in mock- and RA-injected SCC tumours. RA- versus mock-injected tumour comparison has been conducted by using the ΔΔCT method and normalized to glyceraldehyde-3-phosphate dehydrogenase (GAPDH) transcript. Data are represented as mean±s.d. ( n =7). ( e ) qRT–PCR analysis for Wnt target genes in mock- and RA-injected SCC tumours. RA versus mock-injected tumours comparison has been conducted by using the ΔΔCT method and normalized to GAPDH transcript. Data are represented as mean±s.d. ( n =5). ( f ) Immunofluorescence staining for Sox9 in mock- and RA-injected SCC tumours (scale bar, 50 μm). Full size image All together, these data show that forced activation of RA signalling is capable of inducing malignant SCC regression through Wnt inhibition and activation of differentiation programmes. A major challenge in cancer biology is to identify key mechanisms that can be targeted to eradicate the disease. In order to identify such mechanisms, we took advantage of studying self-regressing tumours since they can teach us the physiological mechanisms of tumour regression [5] . Importantly, our self-regressing skin tumour model, keratoacanthoma (KA), provides key advantages over other tumours. Given the skin’s unique accessibility, KA tumours can be easily tracked over time and manipulated, unlike most of the other tumours that affect internal organs. In addition, KAs share cellular origin and signalling mechanisms with more aggressive tumours, such as SCC [39] , [40] , thereby making our discoveries on the self-regressing KA tumours highly relevant towards more aggressive malignant cancers. Here we show that the cellular mechanisms involved in the spontaneous tumour regression include loss of undifferentiated cells and increased differentiation. Thus, HFSC descendants contribute to KA development similarly to what has been found in SCC studies [39] . Remarkably, HFSC-derived cells within the tumours can give rise to both undifferentiated P-cadherin + /Sox9 + cells, consistent with their normal stem cell signature [41] , and differentiated lineages to which they do not normally contribute, such as epidermal differentiated Krt10 + cells [42] . This finding clearly indicates that HFSC descendants are not only capable of adapting to a new environment and modifying their molecular signature, but they are also able to sustain these changes over a long period of time (several months). This is in contrast to other contexts such as epidermal wound for instance, where HFSC descendants are recruited to repair the epidermal wound but get eliminated within few weeks [43] . Notably, stem cell descendant cells and markers of stemness/proliferation (Ki67/Sox9) are dramatically decreased during the regression phase, while instead activation of the differentiation programme takes over. This is quite novel as most current cancer therapeutics are designed to target cancer cell viability [44] . However, in most cases, these approaches have failed to promote long-lasting response suggesting that other cell biological mechanisms in addition to cell proliferation and death may underlie tumour regression [45] . The fact that we clearly demonstrate that regression is driven by differentiation is a key finding and has important therapeutic implication, because it shows that differentiation therapy is possible in solid tumours. Consistent with this rationale, more aggressive tumours have recently been reported to respond well to differentiation therapy, including breast cancer tumours [46] . Developmental programs are often hijacked during cancer. Here we show that developmental and regenerative pathways such as Wnt and RA [47] , [48] , [49] , [50] pathways are re-utilized by KA tumours to drive their spontaneous regression. Wnt is a central mechanism for cancer in several tissues. Wnt activation has been implicated in the initiation, progression and metastasis of different forms of solid tumours, including skin, colon and breast cancer [25] , [26] , [51] , [52] . In skin tumours, Wnt activation drives tumour growth in malignant SCC and melanoma [29] , [53] . In our self-regressing tumour model, Wnt/β-catenin signalling is functionally active during the growth phase but gets downregulated during the regression phase, as we show by several independent lines of evidence in vivo such as nuclear β-catenin, Wnt reporter and Wnt target genes. Strikingly, we demonstrate that Wnt inhibition is sufficient and required for tumour regression both by inhibitor topical delivery and genetic approaches in vivo . While cancer development was predominantly viewed as driven by a cell autonomous mechanism at first, recent evidences have elucidated the role of the tumour microenvironment towards tumour growth [28] , [54] , [55] , [56] . Epithelial/stroma interaction has been shown to play a crucial role in development as well as tissue regeneration [12] , [34] , [57] . In our KA mouse model, we demonstrate that epithelium/stroma signalling cross-talk is important for Wnt regulation. We found that the tumoural epithelium is the source of Wnt ligands, as shown by Wntless and Wnt ligand expression, thus activating Wnt programme and fueling KA growth. Consistent with this, inhibition of Wnt secretion induces reduced proliferation and loss of epithelial cells in our KA model. In contrast, during regression, Wnt inhibitors such as Sfrps are secreted by the stroma and can dampen epithelial Wnt activation thus leading to tumour regression. Overall, these data show the role for Wnt signalling in self-regressing KA tumours, as its temporal activation/inhibition regulation in the epithelium dictates tumour diagnosis. In clinical practice, several retinoid-based drugs have been used for preventing skin tumours. Low levels of RA have been shown to have a tumour-promoting activity [58] . However, the mechanism by which RA acts is unknown [59] , [60] . Our finding of RA acting upstream of Wnt downregulation to trigger tumour regression elucidates the mechanism of action of such drugs. RA upregulation is the key to tumour regression, as shown by our data, because it (1) represents an early event during regression, (2) downregulates the Wnt pathway, (3) decreases proliferation and (4) induces increased differentiation, ultimately leading to tumour regression, in contrast with previous in vitro data showing that RA represses keratinocytes differentiation [61] . Our findings are consistent with examples documented in developmental contexts where RA signalling can inhibit Wnt by inducing the transcription of mesenchymal Wnt inhibitors [38] , [56] , [62] . While initial RA signalling upregulation is observed early during tumour regression, we think that a certain threshold of RA activation is required in order to trigger Wnt downregulation. Here we find that RA activation is followed by upregulation of stromal Wnt inhibitors Sfrp2 and Sfpr4 , which can act on the epithelium to promote cell differentiation and KA tumour regression. Interestingly, our data support that failure of RA activation could result in SCC, as its low expression is comparable with KA tumours during the growth phase. Moreover, we show that RA can induce regression of SCC with a similar signalling cascade observed during KA regression. Thus, this study puts forward a novel molecular mechanism that explains the effect of retinoids on Wnt in a tumoural context in vivo, as shown in Fig. 8 . 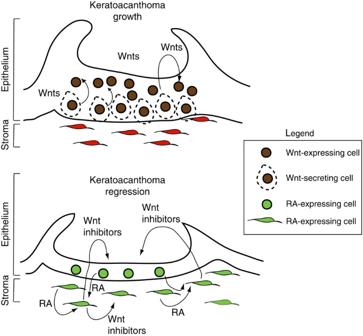Figure 8: A working model of the signalling mechanisms that regulate Keratoacanthoma tumour growth and regression. During Keratoacanthoma tumour growth, Wnt ligands secreted by the epithelium activate the Wnt pathway and sustain tumour growth. During keratoacanthoma regression, the RA signalling pathway is activated in both tumour epithelium and stroma; stromal Wnt inhibitors signal to the epithelium, thus inducing terminal differentiation and regression. Figure 8: A working model of the signalling mechanisms that regulate Keratoacanthoma tumour growth and regression. During Keratoacanthoma tumour growth, Wnt ligands secreted by the epithelium activate the Wnt pathway and sustain tumour growth. During keratoacanthoma regression, the RA signalling pathway is activated in both tumour epithelium and stroma; stromal Wnt inhibitors signal to the epithelium, thus inducing terminal differentiation and regression. Full size image In conclusion, by exploiting in-depth knowledge of the mechanisms that sustain skin regeneration, we have identified key cellular and signalling mechanisms that drive tumour regression by utilizing a self-regressing skin tumour model. Undifferentiated proliferative epithelial cell loss and differentiation are primary drivers for the regression of these tumours along with the novel axis of RA/Wnt-β-catenin regulation that, when targeted, can trigger tumour regression. Importantly, these findings are highly relevant in the cancer field, because they provide potential therapeutic strategies for other Wnt-dependent skin malignant tumours that do not self-regress spontaneously, such as SCCs. Generation of experimental mice K19Cre ER knock in mice, K14Cre, K14Cre ER , TcfLef-H2BGFP and Rosa26mTmGFP (GFPr) transgenic mice have been used to label respectively, the HFSCs, the epithelial cells and the Wnt-responsive cells within KA tumours [30] , [32] , [36] , [63] . K19Cre ER ; Rosa26mTmGFP , K14Cre ; Rosa26mTmGFP and K14Cre ER ; Rosa26mTmGFP ; β -catn flox(Ex3)/+ have been generated and mouse genotyping has been performed by PCR. Eight-week-old male and female mice have been used for the induction of skin tumours, DMBA based. All the experiments have been conducted on littermate mice obtained from the same breeding. K19Cre ER ; Rosa26mTmGFP were induced with 1 mg of tamoxifen (Sigma) every day for 10 consecutive days starting at postnatal day 44 (second hair follicle rest phase) to label HFSCs. K14Cre ER ; Rosa26mTmGFP ; β -catn flox(Ex3)/+ and control littermates K14Cre ER ; Rosa26mTmGFP were induced with 1 mg of tamoxifen (Sigma) every day for 5 consecutive days starting at 16 weeks post-DMBA treatment. Chemical carcinogenesis protocol and tumour pathology Carcinogenesis protocol has been performed as previously shown [11] , [64] , [65] . Briefly, 7-week-old mice have been treated with 25 μg of DMBA (D32-54-1G, Sigma) twice a week for up to 20 weeks. To obtain SCCs, DMBA treatment was continued up to 24 weeks. To assess KA self-regression, DMBA has been stopped at 16th week and mice were maintained up to 8 weeks post DMBA. Mice were monitored weekly for assessing tumour number, appearance and size. Tumour histology was analysed by the dermatopathologist Dr Christine Ko (Yale, Department of Dermatology). All the studies are approved by the IACUC committee and followed NIH guidelines. Tissue harvesting DMBA-induced mouse tumours were harvested and processed for RNA extraction, paraffin and optimum cutting temperature (OCT) compound embedding. Briefly, for RNA extraction, the tumour specimen has been flash frozen in liquid nitrogen and then stored at −80 °C for next use. For paraffin embedding, each tumour has been fixed overnight in 10% formalin and then processed by the Dermatopathology laboratory at Yale University. For OCT embedding, tumour samples were incubated in OCT for 1 h at 4 °C before embedding. In vivo and in vitro Wnt inhibitor and RA treatments Wnt inhibitor IWP2 has been obtained from Stemgent. IWP2 was reconstituted in dimethylsulphoxide and diluted in phosphate-buffered saline (PBS) to obtain a 50 μM working solution in 20 μl of injected volume. Mice tumours have been injected with IWP2 for 7 days consecutively starting at 16 weeks of DMBA treatment. The same experimental protocol has been used for RA treatment of both KAs and SCCs (R2625-500 mg, Sigma) (100 μM working solution in 20 μl of injected volume). Tumours have been harvested at 2 days and 4 weeks post IWP2 and RA treatment. For in vitro experiments, wild-type keratinocytes were treated with 10 μM RA for 1 and 4 days. At the end of each experimental time point, the cells were collected for RNA extraction with the RNeasy Plus Mini Kit (74134, Qiagen). RNA analyses RNA from whole tumour tissue has been isolated with RNeasy Fibrous Tissue Mini Kit (74704, Qiagen), according to the manufacturer’s instruction. Similarly, for FACS-isolated tumour cells, RNA was extracted by using RNeasy Plus Mini Kit (Qiagen). RNA was retrotranscribed into cDNA by using Superscript III First-Strand Synthesis System (18080-051, Life Technologies). qRT–PCR reactions have been performed by using ViiA7 Real-Time Machine System (Applied Biosystem). A total of 5 ng of cDNA was used for each reaction with Fast Start SYBR Green Master Mix (Roche). The list of all primers used is reported in Supplementary Table 2 . Gene expression analysis has been conducted using the ΔΔCT method and utilizing glyceraldehyde-3-phosphate dehydrogenase as housekeeping gene. Flow cytometry and FACS Growing and regressing KAs and SCC tumours were dissected out and rinsed with PBS. A portion was devoted to histology and the rest digested for single-cell suspension. For the latter, each tumour was minced in 2.5 mg ml −1 collagenase (Sigma) with a razor blade and incubated at 37 °C for 50 min. After mechanical dissociation, 0.25% Trypsin (Life Technologies) was added and the cell suspension was incubated at 37 °C for 5 min. Wash solution (4% fetal bovine serum in PBS) was added to stop the reaction, followed by pipetting up and down to make single-cell suspension. Single cells were filtered through 40 micron strainer and then readied for staining with surface antibodies. To isolate HFSCs, subcutaneous fat was removed from the skin and placed on Hank’s balanced salt solution containing 0.2% collagenase (Sigma) for 30 min at 37 °C. The remaining tissue after digestion was then treated with Trypsin (Gibco) at 37 °C for additional 30 min. Skin cell suspension was eventually collected and filtered through strainers (70 μm, the 40-μm pores, BD Biosciences). For FACS analysis, single-cell suspension in 2% fetal bovine serum in PBS was exposed to the appropriate conjugated antibody for 15 min at 4 °C. The list of the antibodies used for the isolation of HFSCs is shown in Supplementary Table 3 . FACS profiles have been analysed through the FlowJo software. Immunostaining on paraffin and frozen sections After rehydration, paraffin-embedded tumour sections have been subjected to antigen retrieval with 10 mM citrate buffer pH 6.0 and then incubated overnight at 4 °C with primary antibodies at concentrations listed in Supplementary Table 3 . For mouse antibodies, the M.O.M. kit was used (Vector Laboratories). β-Catenin immunohistochemistry has been conducted as previously described [16] . Secondary antibodies conjugated with FITC, RRX and Cy5 (Jackson Immunoresearch Laboratories) were used at a concentration of 1:100 for 1 h at room temperature. Slides were mounted with Vectashield Mounting Media with 4′,6-diamidino-2-phenylindole (H-1200, Vector Laboratories). For cryosection immunostaining, 10-μm sections from skin tumour samples were fixed in paraformaldehyde for 10 min at room temperature and the dilutions used for the immunostainings are indicated in the Supplementary Table 3 . Secondary antibodies have been used as described above. In situ hybridization on frozen tissue sections In situ hybridization was performed according to standard protocols using DIG-labelled antisense riboprobes [66] . Wnt3 riboprobe was made by PCR from RNA extracted from mouse back skin (forward primer: 5′-gctcctttggtaccagggac-3′; reverse primer: 5′-tcgccatggtcttgtccttc-3′). A total of 10 μm skin sections were fixed in 4% PFA and counterstained with DAPI. RNA sequencing RNA samples from KAs at 0 and 1 week post-DMBA treatment were sequenced on a HiSeq 2000 (Illumina, San Diego, CA, USA). The original 75 bp pair-ended reads were preprocessed with Trimmomatic [67] (version 0.30) to trim off the adaptor sequence and poorly scored base pairs. The processed reads were then aligned to the mouse transcriptome (mm9) with Tophat [68] (version 2.0.8) and the numbers of reads uniquely and unanimously mapped to each annotated gene (mm9) were counted with HTSeq-count (version 0.5.4, http://www-huber.embl.de/users/anders/HTSeq ). The differentially expressed genes were detected using EdgeR [69] (version 3.3.3), cutting off a P- value less than 0.001 based on the negative binomial distribution of the count data. The data have been deposited in NCBI’s Gene expression Omnibus, and are accessible through GEO Series accession number GSE54098 ( http://www.ncbi.nlm.nih.gov/geo/query/acc.cgi?acc=GSE54098 ). Statistical analysis Data are expressed as mean±s.d. An unpaired Student's t -test was used to analyse data sets with two groups. For all analyses, P<0.05 was accepted as indicating a significant difference. Statistical calculations were performed using the Prism software package (GraphPad, USA). Accession codes : The mRNA-seq data have been deposited in the Gene expression Omnibus database under accession code GSE54098 . How to cite this article : Zito, G. et al. Spontaneous tumour regression in keratoacanthomas is driven by Wnt/retinoic acid signalling cross-talk. Nat. Commun. 5:3543 doi: 10.1038/ncomms4543 (2014).